All-organic optoelectronic sensor for pulse oximetry Pulse oximetry is a ubiquitous non-invasive medical sensing method for measuring pulse rate and arterial blood oxygenation. Conventional pulse oximeters use expensive optoelectronic components that restrict sensing locations to finger tips or ear lobes due to their rigid form and area-scaling complexity. In this work, we report a pulse oximeter sensor based on organic materials, which are compatible with flexible substrates. Green (532 nm) and red (626 nm) organic light-emitting diodes (OLEDs) are used with an organic photodiode (OPD) sensitive at the aforementioned wavelengths. The sensor’s active layers are deposited from solution-processed materials via spin-coating and printing techniques. The all-organic optoelectronic oximeter sensor is interfaced with conventional electronics at 1 kHz and the acquired pulse rate and oxygenation are calibrated and compared with a commercially available oximeter. The organic sensor accurately measures pulse rate and oxygenation with errors of 1% and 2%, respectively. Conventional pulse oximeters non-invasively measure human pulse rate and arterial blood oxygen saturation with an optoelectronic sensor composed of two inorganic light-emitting diodes (LEDs) with different peak emission wavelengths and a single inorganic photodiode [1] , [2] . The LEDs are placed on one side of a finger and the light transmitted through the tissue is subsequently sensed by the photodiode that is placed on the opposite side of the finger. Sequential sampling of the transmitted light provides information on the ratio of oxygenated and deoxygenated haemoglobin in the blood. This ratio and a calibration curve are used to compute arterial blood oxygen saturation. Currently, the application of commercially available pulse oximeters is limited by the bulk, rigidity and high large-area scaling cost of conventional inorganic-based optoelectronics. Here we show a pulse oximeter sensor composed of organic LEDs (OLEDs) [3] , [4] and a flexible organic polymer photodiode (OPD) [5] . We successfully demonstrate that the organic optoelectronic sensor provides accurate measurement capability and we anticipate that our application of solution-processable organic optoelectronics in pulse oximetry will enable low-cost, disposable and wearable medical devices. Wearable medical sensors have the potential to play an essential role in the reduction of health care costs: they encourage healthy living by providing individuals feedback on personal vital signs and enable the facile implementation of both in-hospital and in-home professional health monitoring. Consequently, wide implementation of these sensors can reduce prolonged hospital stays and cut avertible costs [6] . Recent reports show ample wearable sensors capable of measuring pressure [7] , [8] , biopotential and bioimpedance [9] , [10] , pulse rate [11] and temperature [12] , [13] in real time. These sensors are developed in wearable and flexible form factors using organic [8] , [13] , [14] , inorganic [12] , [15] , [16] and hybrid organic–inorganic [7] , [9] , [15] materials. Organic semiconductors developed for OLEDs and OPDs have been primarily applied to display and photovoltaic technologies [17] , [18] . This is due to their potential for large-area roll-to-roll manufacturing at large volumes, which is enabled by solution processing and the use of flexible substrates [19] . These attributes also make organic optoelectronics very attractive for medical sensors, where flexibility combined with large areas can result in an improvement of the overall sensor performance. In the past 10 years, a lot of resources were used to improve the stability of organic semiconductors to meet the lifetime requirements of displays and photovoltaics [20] , [21] . When compared with the above markets, disposable medical sensors have less-stringent lifetime requirements on the materials, since these devices would be used only for a few days as opposed to years. Indeed, organic optoelectronics have previously been used to perform pulse measurements [22] , [23] , [24] . Here we report a sensor composed solely of organic optoelectronics that measures both human pulse and arterial blood oxygenation. We anticipate that our results will inspire system-level integration of organic–inorganic electronics, where the large area, low cost and mechanical flexibility of organic sensors will be combined with the computational efficiency of inorganic electronics. A schematic view of the sensor is given in Fig. 1a , where two OLED arrays and two OPDs are placed on opposite sides of a finger. 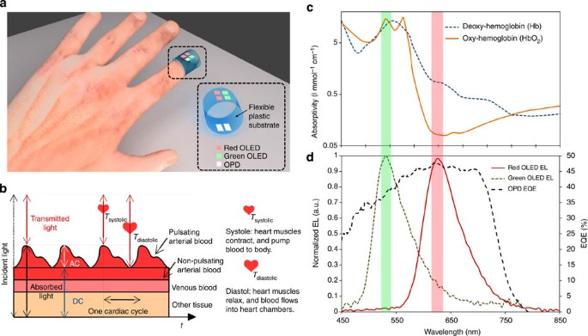Figure 1: Pulse oximetry with an organic optoelectronic sensor. (a) Pulse oximetry sensor composed of two OLED arrays and two OPDs. (b) A schematic illustration of a model for the pulse oximeter’s light transmission path through pulsating arterial blood, non-pulsating arterial blood, venous blood and other tissues over several cardiac cycles. The a.c. and d.c. components of the blood and tissue are designated, as well as the peak and trough of transmitted light during diastole (Tdiastolic) and systole (Tsystolic), respectively. (c) Absorptivity of oxygenated (orange solid line) and deoxygenated (blue dashed line) haemoglobin in arterial blood as a function of wavelength. The wavelengths corresponding to the peak OLED electroluminescence (EL) spectra are highlighted to show that there is a difference in deoxy- and oxy-haemoglobin absorptivity at the wavelengths of interest. (d) OPD EQE (black dashed line) at short circuit, and EL spectra of red (red solid line) and green (green dashed line) OLEDs. Figure 1: Pulse oximetry with an organic optoelectronic sensor. ( a ) Pulse oximetry sensor composed of two OLED arrays and two OPDs. ( b ) A schematic illustration of a model for the pulse oximeter’s light transmission path through pulsating arterial blood, non-pulsating arterial blood, venous blood and other tissues over several cardiac cycles. The a.c. and d.c. components of the blood and tissue are designated, as well as the peak and trough of transmitted light during diastole ( T diastolic ) and systole ( T systolic ), respectively. ( c ) Absorptivity of oxygenated (orange solid line) and deoxygenated (blue dashed line) haemoglobin in arterial blood as a function of wavelength. The wavelengths corresponding to the peak OLED electroluminescence (EL) spectra are highlighted to show that there is a difference in deoxy- and oxy-haemoglobin absorptivity at the wavelengths of interest. ( d ) OPD EQE (black dashed line) at short circuit, and EL spectra of red (red solid line) and green (green dashed line) OLEDs. Full size image Pulse and oxygenation with red and green organic light emitting diodes In contrast to commercially available inorganic oximetry sensors, which use red and near-infrared LEDs, we use red and green OLEDs. Incident light from the OLEDs is attenuated by pulsating arterial blood, non-pulsating arterial blood, venous blood and other tissue as depicted in Fig. 1b . When sampled with the OPD, light absorption in the finger peaks in systole (the heart’s contraction phase) due to large amount of fresh arterial blood. During diastole (the heart’s relaxation phase), reverse flow of arterial blood to the heart chambers reduces blood volume in the sensing location, which results in a minima in light absorption. This continuous change in arterial blood volume translates to a pulsating signal—the human pulse. The d.c. signal resulting from the non-pulsating arterial blood, venous blood and tissue is subtracted from the pulsating signal to give the amount of light absorbed by the oxygenated and deoxygenated haemoglobin in the pulsating arterial blood. Oxy-haemoglobin (HbO 2 ) and deoxy-haemoglobin (Hb) have different absorptivities at red and green wavelengths, as highlighted on the absorptivity of oxygenated and deoxygenated haemoglobin plotted in Fig. 1c . The difference in the molar extinction coefficient of oxygenated and deoxygenated haemoglobin at the green wavelength is comparable to the difference at near-infrared wavelengths (800–1,000 nm) used in conventional pulse oximeters. In addition, solution-processable near-infrared OLED materials are not stable in air and show overall lower efficiencies [25] , [26] . Thus, we elected to use green OLEDs instead of near-infrared OLEDs. Using red and green OLEDs and an OPD sensitive at visible wavelengths (the OLEDs’ emission spectra and the OPD’s external quantum efficiency (EQE) as a function of incident light wavelength are plotted in Fig. 1d ), blood oxygen saturation (SO 2 ) is quantified according to equation 1. Here, and C Hb are the concentrations of oxy-haemoglobin and deoxy-haemoglobin, respectively. R os , the ratio of absorbed red ( A rd ) and green ( A gr ) light, depends on the normalized transmitted red ( T n,rd ) and green ( T n,gr ) light intensities according to Beer–Lambert’s law (shown in equation 2). Finally, arterial oxygen saturation (S a O 2 ) can be calculated using equation 3. Here, ε rd,Hb and ε gr,Hb are the molar absorptivity of deoxy-haemoglobin at red ( λ =626 nm) and green ( λ =532 nm) wavelengths, respectively. Similarly, and are the molar absorptivity of oxy-haemoglobin at red ( λ =626 nm) and green ( λ =532 nm) wavelengths, respectively. Organic optoelectronic oximeter components OLED and OPD performances are both paramount to the oximeter measurement quality. The most important performance parameters are the irradiance of the OLEDs' ( Fig. 2b ) and the EQE at short circuit of the OPD ( Figs 1d and 3b ). As the OLEDs operating voltage increases, irradiance increases at the expense of efficiency [27] , as shown by the lower slope of irradiance than current as a function of applied voltage in Fig. 2b . For a pulse oximeter, this is an acceptable trade-off because higher irradiance from the OLEDs yields a strong measurement signal. 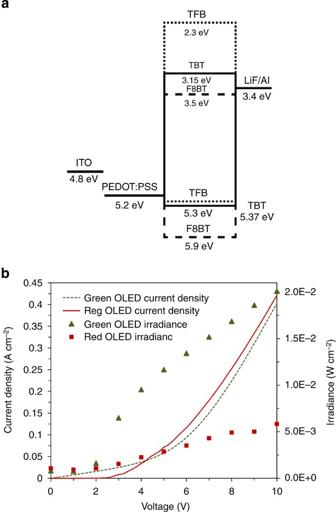Figure 2: OLED design and performance. (a) OLED energy structure. (b) Current density of red (red solid line) and green (green dashed line) OLEDs and irradiance of red (red squares) and green (green triangles) OLEDs as a function of applied voltage. Figure 2: OLED design and performance. ( a ) OLED energy structure. ( b ) Current density of red (red solid line) and green (green dashed line) OLEDs and irradiance of red (red squares) and green (green triangles) OLEDs as a function of applied voltage. 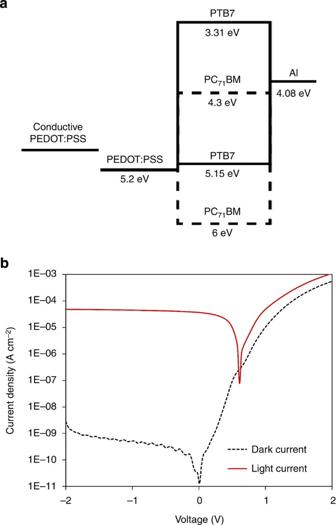Figure 3: OPD design and performance. (a) OPD energy structure. (b) Light current (red solid line) with excitation from a 640 nm, 355 μW cm−2light source and dark current (black dashed line) as a function of applied voltage. Full size image Figure 3: OPD design and performance. ( a ) OPD energy structure. ( b ) Light current (red solid line) with excitation from a 640 nm, 355 μW cm −2 light source and dark current (black dashed line) as a function of applied voltage. Full size image We have selected polyfluorene derivatives as the emissive layer in our OLEDs due to their environmental stability, relatively high efficiencies and self-assembling bulk heterojunctions that can be tuned to emit at different wavelengths of the light spectrum [4] . The green OLEDs were fabricated from a blend of poly(9,9-dioctylfluorene- co -n-(4-butylphenyl)-diphenylamine) (TFB) and poly((9,9-dioctylfluorene-2,7-diyl)-alt-(2,1,3-benzothiadiazole-4,8-diyl)) (F8BT). In these devices, electrons are injected into the F8BT phase of phase-separated bulk-heterojunction active layer while holes are injected into the TFB phase, forming excitons at the interfaces between the two phases and recombining in the lower energy F8BT phase for green emission [28] . The emission spectrum of a representative device is shown in Fig. 1d . The red OLED was fabricated from a tri-blend blend of TFB, F8BT and poly((9,9-dioctylfluorene-2,7-diyl)-alt-(4,7-bis(3-hexylthiophene-5-yl)-2,1,3-benzothiadiazole)-2′,2′-diyl) (TBT) with an emission peak of 626 nm as shown in Fig. 1d . The energy structure of the full stack used in the fabrication of OLEDs, where ITO/PEDOT:PSS is used as the anode, TFB as an electron-blocking layer [29] and LiF/Al as the cathode, is shown in Fig. 2a . The physical structure of the device is provided in Supplementary Fig. 2b . The red OLED operates similarly to the green, with the additional step of excitonic transfer via Förster energy transfer [30] to the semiconductor with the lowest energy gap in the tri-blend, TBT, where radiative recombination occurs. The irradiance at 9 V for both types of OLEDs, green and red, was measured to be 20.1 and 5.83 mW cm −2 , respectively. The ideal OPD for oximetry should exhibit stable operation under ambient conditions with high EQE at the peak OLED emission wavelengths (532 and 626 nm). A high EQE ensures the highest possible short-circuit current, from which the pulse and oxygenation values are derived. Poly({4,8-bis[(2-ethylhexyl)oxy]benzo[1,2- b :4,5-b′]dithiophene-2,6-diyl}{3-fluoro-2-[(2-ethylhexyl)carbonyl]thieno[3,4–b]thiophenediyl}) (PTB7) mixed with [6,6]-phenyl C71-butyric acid methyl ester (PC 71 BM) is a stable donor:acceptor bulk-heterojunction OPD system, which yields EQE as high as 80% for spin-coated devices [5] . The transparent electrode and active layer of the OPD are printed on a plastic substrate using a surface tension-assisted blade-coating technique recently developed and reported by Pierre et al . [31] Figure 3a shows the energy band structure of our device including the transparent electrode (a high-conductivity/high-work-function PEDOT:PSS bilayer) and an Al cathode. The physical device structure of the OPD is shown in Supplementary Fig. 2d . The EQE at 532 and 626 nm is 38 and 47%, respectively, at short-circuit condition, as shown in Fig. 1d , and the leakage current of about 1 nA cm −2 at 2 V applied reverse bias is shown in Fig 3b together with the photocurrent when the device is illuminated with a 355 μW cm −2 light source at 640 nm. Despite the low reverse bias leakage current shown in Fig 3b , we chose to bias the OPD at 0 V, the short-circuit condition, to sense low photocurrent levels. The frequency response of both the OPD and OLEDs was also characterized, since oximetry is usually performed at 1 kHz. The 3 dB cut-off was found to be at frequencies higher than 10 kHz for the all-organic optoelectronic sensor, which is significantly higher than the operational frequency required for oximetry ( Supplementary Fig. 4 ). Notably, the frequency performance of the OPD is not hampered at short circuit because the shunt capacitance of organic photodiodes decreases negligibly with reverse bias, unlike inorganic photodiodes [32] . We observed that the OLED irradiance for both red and green wavelengths is sufficient for the transmission of light through the finger and the signal acquired by the organic photodetector is sufficiently high for resolving the pulsating photoplethysmogram (PPG) signal shown in Fig. 1b . The pulse waveforms (two cardiac cycles) generated with a combination of organic and inorganic devices are shown in Fig. 4 . The PPG obtained when a human finger is illuminated by inorganic LEDs and the transmitted light is measured with an OPD is shown in Fig. 4a . When the same measurement is performed using OLEDs and a conventional Si photodiode ( Fig. 4b ), the magnitude of the PPG signal is reduced from 26 to 16 mVp-p for the green and 16 to 6 mVp-p for the red due to the lower optical power of the organic LEDs compared with their inorganic equivalent device. Finally, both OLEDs and an OPD are used to obtain a PPG under the same experimental conditions ( Fig. 4c ), yielding signal magnitudes of 3 mVp-p for the green and 2.5 mVp-p for the red. It is clear that the magnitude of the signal is substantially reduced with the introduction of organic-based devices, but the PPG obtained at red and green wavelengths yields similar shapes for all device combinations shown in Fig. 4 , which will result in similar pulse and arterial oxygenation values. The lower signal magnitude shown by the organic probe is compensated for by increasing the area of devices, resulting in higher photocurrents that directly translate into higher PPG signals, as shown in Supplementary Fig. 3a . 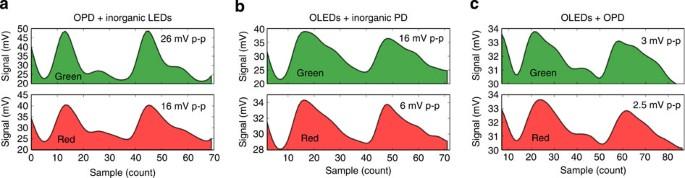Figure 4: PPG acquisition using combinations of inorganic and organic LEDs and photodiodes (PDs). (a) PPG signal acquired using inorganic red and green LEDs and an OPD. Green and red PPG signal amplitudes of 26 and 16 mVp-p were obtained, respectively. (b) PPG signal acquired using OLEDs and silicon PD—absence of lensing epoxy and reduced irradiance of the OLEDs bring down signal magnitude to 16 and 6 mVp-p for green and red excitations. (c) PPG signal acquired using OLEDs and OPD; although signal magnitudes are reduced to 3 and 2.5 mVp-p, the signal is sufficient for resolving the PPG waveform and provide light absorbance ratio information for arterial blood oxygenation calculation. Figure 4: PPG acquisition using combinations of inorganic and organic LEDs and photodiodes (PDs). ( a ) PPG signal acquired using inorganic red and green LEDs and an OPD. Green and red PPG signal amplitudes of 26 and 16 mVp-p were obtained, respectively. ( b ) PPG signal acquired using OLEDs and silicon PD—absence of lensing epoxy and reduced irradiance of the OLEDs bring down signal magnitude to 16 and 6 mVp-p for green and red excitations. ( c ) PPG signal acquired using OLEDs and OPD; although signal magnitudes are reduced to 3 and 2.5 mVp-p, the signal is sufficient for resolving the PPG waveform and provide light absorbance ratio information for arterial blood oxygenation calculation. Full size image System design for an organic optoelectronic pulse oximeter The organic pulse oximetry sensor composed of two red and green OLED arrays and an OPD ( Fig. 5a ) is interfaced with a microcontroller that drives the OLEDs, measures the OPD signal and transfers the data to a computer for analysis ( Fig. 5b ). The obtained signal from the OPD passes through an analogue front end where the PPG signal is filtered and amplified. The pulsating part of the signal yields heart rate and oxygenation according to an empirical correction to equation 3 (details are provided in Supplementary Methods and Supplementary Fig. 1 ). The accuracy of the organic optoelectronic sensor is characterized and calibrated by comparing pulse and oxygenation measurements taken simultaneously by the organic optoelectronic sensor and a commercially available pulse oximeter. The resultant pulse waveforms, pulse value, ratio of absorbed light and arterial blood oxygen saturation from the red and near-infrared LEDs in the inorganic oximeter and the red and green OLEDs in the organic oximeter are shown in Fig. 5c,d , respectively. The OLEDs are powered by a 9 V battery and the OPD is biased at 0 V. The a.c. component of the signal ( Fig. 1b ) is essential for visualizing cardiac rhythm and computing arterial blood oxygen saturation. The OPD read-out circuit consists of two internal operational amplifiers ( Fig. 5b ) in which the first stage amplifies the whole PPG signal from the photodiode. The second stage only amplifies the pulsating part of the signal and is read by an analogue-to-digital converter (ADC). With two-stage amplification, we obtained a 50–60 mVp-p PPG signal for the inorganic probe ( Fig. 5c ) and a 3–4 mVp-p PPG signal for the organic probe ( Fig. 5d ). The heart rate and ratio of transmitted light at two wavelengths ( Fig. 5c,d ) were calculated directly from the PPG signals and the arterial blood oxygen saturation was derived from the ratio of transmitted light, as discussed previously and in the Supplementary Methods . The calculated heart rate and oxygenation derived from the PPG signals from the inorganic and organic probes are both 65–70 beats per minute and 94–96%, respectively ( Fig. 5c,d ). We observed 1% error for pulse rate and 2% error for oxygenation when comparing the organic optoelectronic sensor with the inorganic sensor. 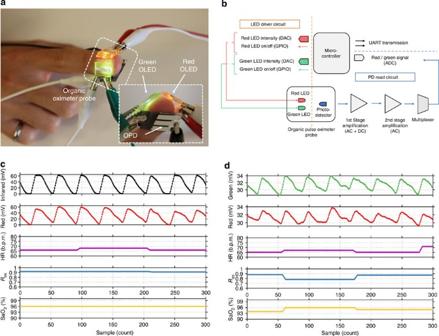Figure 5: Organic optoelectronic pulse oximetry system. (a) Red and green OLEDs are placed on subject’s finger and transmitted light is collected with one OPD pixel placed below the finger. (b) Hardware block diagram for the system set-up—a microcontroller acts as the data acquisition and processing unit. OLEDs are triggered and controlled using general-purpose input/output port and DAC pins, and the OPD signal is recorded using the ADC of the microcontroller. A two-stage amplifier between the OPD and ADC removes the d.c. part from the PPG signal and amplifies the pulsating PPG signal. (c,d) Simultaneous oximetry measurements with a commercially available inorganic oximeter probe and the organic oximeter probe, respectively. The PPG signal was obtained using red and infrared light for the commercially available probe (c) and using red and green light for the organic probe (d). Heart rate (HR; magenta line inc,d) was obtained by timing the systolic peaks in the PPG signals. The ratio of the transmitted light at two wavelengths (Ros; blue line inc,d) is converted to arterial blood oxygen saturation (SaO2; yellow line inc,d) using Beer–Lambert’s law in conjunction with an empirical correction. Figure 5: Organic optoelectronic pulse oximetry system. ( a ) Red and green OLEDs are placed on subject’s finger and transmitted light is collected with one OPD pixel placed below the finger. ( b ) Hardware block diagram for the system set-up—a microcontroller acts as the data acquisition and processing unit. OLEDs are triggered and controlled using general-purpose input/output port and DAC pins, and the OPD signal is recorded using the ADC of the microcontroller. A two-stage amplifier between the OPD and ADC removes the d.c. part from the PPG signal and amplifies the pulsating PPG signal. ( c , d ) Simultaneous oximetry measurements with a commercially available inorganic oximeter probe and the organic oximeter probe, respectively. The PPG signal was obtained using red and infrared light for the commercially available probe ( c ) and using red and green light for the organic probe ( d ). Heart rate (HR; magenta line in c , d ) was obtained by timing the systolic peaks in the PPG signals. The ratio of the transmitted light at two wavelengths ( R os ; blue line in c , d ) is converted to arterial blood oxygen saturation (S a O 2 ; yellow line in c , d ) using Beer–Lambert’s law in conjunction with an empirical correction. Full size image Motion artefacts are one possible source of error in pulse oximetry measurements. Motion-induced errors can be minimized with signal-processing algorithms that can be found in literature [33] , [34] . In this work, we focus mainly on organic optoelectronic probe design and development; motion artefact characterization and mitigation algorithms can be implemented to further improve sensor performance. The novel combination of red and green OLEDs, as opposed to a red and near-infrared LED pair, is successfully implemented in pulse oximetry because the difference in the absorptivity of oxygenated and deoxygenated haemoglobin at the green wavelength is comparable to the difference at near-infrared wavelengths [35] as seen in Fig. 1c . Green LEDs have not been used conventionally in transmission oximetry because shorter wavelengths are more efficiently absorbed by the blood. However, the higher irradiance of the green OLEDs ( Fig. 2b ) compensates for any absorption losses in non-pulsating blood and tissue, as can be inferred from the higher green signal amplitudes in Fig. 4 compared with the red signal amplitudes. We employed an empirical correction to calculate arterial blood oxygenation from the ratio of transmitted green and red light, a scheme widely used for correcting for the deviation from Beer–Lambert’s law (which does not account for the scattering that occurs in human tissue) in red and near-infrared pulse oximetry measurements. Aside from maximizing OPD EQE and short-circuit photocurrent and OLED irradiance, the OPD’s short-circuit current resulting from ambient light should be minimized to achieve the best pulse oximetry signal, as parasitic photodetector current is a contributor to conventional pulse oximetry failure [36] . The effects of ambient light on the OPD’s short-circuit current were measured using two-finger phantoms with radii of 9 and 5 mm, representative of the wide range of human finger sizes. Flexing the photodiode around the finger phantom, as opposed to taking the measurement with the photodiode placed flat, non-flexed, against the phantom, significantly reduces the parasitic short-circuit current produced by ambient light. Under typical room-lighting conditions of 72–76 μW cm −2 , flexing the OPD around the 9 and 5 mm radii phantoms reduced the parasitic current from 270 to 20 nA and 280 to 60 nA, respectively ( Supplementary Fig. 3b ). The ability of the flexible OPD to conform around the human body therefore improves the pulse oximeter’s versatility. The long-term stability of the organic optoelectronic pulse oximeter, like most organic optoelectronics, is limited by the robustness of the encapsulation technology employed in its fabrication [37] , [38] . It has been shown that lifetime of organic optoelectronics can be significantly improved using robust encapsulation and packaging. With our encapsulation process, we see a 24% signal intensity decrease in the green and a 54% decrease in the red PPG signal over a 7-day time frame. Supplementary Figure 5 shows a decline in signal intensity; however, the PPG signal shapes are intact. The organic optoelectronic pulse oximetry sensor described here demonstrates the potential for the application of organic electronics to thrive in the medical device field. The large-area scalability, inexpensive processing and flexibility of organic optoelectronics will allow medical sensors to be made in new shapes and sizes, diversifying possible sensing locations on the human body, enabling medical professionals to better monitor their patients’ care. OLED fabrication and characterization The semiconducting polymers used in the emissive layer of the OLEDs were supplied by Cambridge Display Technology Limited. The red OLED active layer was made from a 25:70:5 blend of TFB:F8BT:TBT in a 10 mg ml −1 o -xylene solution. The green OLED active layer was made from a 1:9 blend of TFB:F8BT in a 10 mg ml −1 o -xylene solution. Patterned ITO substrates were cleaned via sonication in acetone and then isopropyl alcohol. The substrate surfaces were made hydrophilic with a 2 min plasma treatment before spincoating a 40 nm layer of Clevios PEDOT:PSS AI4083. Any remaining moisture was evaporated in a 10 min annealing step at 120 °C before moving the samples into a nitrogen glove box for the remainder of the fabrication procedure. TFB was spin coated from a 10 mg ml −1 o -xylene solution and then annealed at 180 °C for 45 min before cooling and spin rinsing with o -xylene, producing a 10–20 nm-thick electron-blocking layer. The active layer was then spun at 4500, r.p.m. for a 100 nm film thickness. The LiF (1 nm)/Al (100 nm) cathode was thermally evaporated under vacuum at 4 × 10 −6 Torr. Finished devices were encapsulated with ultraviolet-curable Delo Katiobond LP612 epoxy and clean quartz glass. Each OLED pixel had 4 mm 2 of active area. OLED current/voltage characteristics and irradiance measurements were taken with an Orb Optronix light measurement system complete with an Orb Optronix SP-50 spectrometer, integrating sphere, Keithley 2400 Source Meter and Spectral Suite 3.0 software. OPD fabrication and characterization OPDs were printed on top of planarized polyethylene naphthalate (PEN) substrates (DuPont) using a blade-coating technique previously reported [31] . A layer of high-conductivity PEDOT:PSS (Sigma-Aldrich, 739316-25G) was printed by blade coating (200 μm blade height at 1.6 cm s −1 ) the solution over a large hydrophilic strip in the substrate defined by a 10 s plasma treatment through a stencil. Following a 10 min anneal at 120 °C, a layer of high-work-function PEDOT:PSS (Clevios Al4083) was coated and annealed over the previous print using the same process. The active layer ink comprised of a 1:1 weight ratio of PTB7:PC 71 BM (Solaris Chem) dissolved to 35 mg ml −1 in chlorobenzene with a 3 vol.% concentration of 1,8-diiodooctane and was blade coated (350 μm blade height at 1.6 cm s −1 ) in a glove box with the substrate heated to 40 °C. The aluminum cathode (100 nm) was thermally evaporated under vacuum at 4 × 10 −6 Torr to yield an active area of 21 mm 2 . Finished devices were encapsulated with ultraviolet-curable Delo Katiobond LP612 epoxy and Saran wrap after being post-annealed at 120 °C for 10 min. All OLED and OPD layer thicknesses were measured with a Dektak Profilometer. Electronic hardware and software for data acquisition and processing The Texas Instruments MSP430 microcontroller was chosen for data acquisition and processing because of its built-in ADCs and digital-to-analogue converters (DACs), which are required for the pulse oximeter. General-purpose input–output pins from the microcontroller control LED switching, ADCs are utilized to read the amplified OPD signal from the multiplexer, and DACs are used to control LED intensity and in the signal amplification stage. The LEDs are operated in a sequential approach, so that only one of the LEDs is on at a particular moment. Five hundred and twelve samples are taken from each of the LEDs per second. A software trigger from the microcontroller controls a PNP bipolar junction transistor (BJT) switch that triggers the LED on/off. In addition, DACs are used to control the drive current for the LEDs using a NPN transistor. For ensuring compatibility with the organic LEDs, signals from the microcontroller are shifted to 9 V using general-purpose operational amplifiers. Finally, universal asynchronous receiver/transmitter (UART) protocol is used to send processed data to a computer for visualization. We opted for a modular approach by separating the LED driver circuit and OPD read circuit, simplifying circuit design and debugging. Hamamatsu Large Area Photodiode S1227-1010BQ (active area of 35 mm 2 ) and 5 mm red and green round LEDs were used in PPG data comparisons with the organic devices. All-pulse oximetry experiments performed on human subjects were carried out with informed consent under the approval of the University of California, Berkeley Institutional Review Board, protocol ID number 2013-03-6081. How to cite this article : Lochner, C. M. et al . All-organic optoelectronic sensor for pulse oximetry. Nat. Commun. 5:5745 doi: 10.1038/ncomms6745 (2014).